Rapid cell-surface prion protein conversion revealed using a novel cell system Prion diseases are fatal neurodegenerative disorders with unique transmissible properties. The infectious and pathological agent is thought to be a misfolded conformer of the prion protein. Little is known about the initial events in prion infection because the infecting prion source has been immunologically indistinguishable from normal cellular prion protein (PrP C ). Here we develop a unique cell system in which epitope-tagged PrP C is expressed in a PrP knockdown (KD) neuroblastoma cell line. The tagged PrP C , when expressed in our PrP-KD cells, supports prion replication with the production of bona fide epitope-tagged infectious misfolded PrP (PrP Sc ). Using this epitope-tagged PrP Sc , we study the earliest events in cellular prion infection and PrP misfolding. We show that prion infection of cells is extremely rapid occurring within 1 min of prion exposure, and we demonstrate that the plasma membrane is the primary site of prion conversion. Transmissible spongiform encephalopathies or prion diseases are fatal neurodegenerative diseases of humans and animals, and are characterized by the accumulation of misfolded prion protein (PrP Sc ) in the brain [1] . Prion disease is caused by the templated misfolding of a normal host cellular prion protein (PrP C ) by PrP Sc , which can be derived either by infection from an exogenous prion source (for example, scrapie in sheep, bovine spongiform encephalopathy in cattle and kuru in humans), from the pathological misfolding of endogenous PrP C due to mutations in the PrP gene (for example, fatal familial insomnia) or due to rare stochastic misfolding of normal PrP C protein (for example, sporadic Creutzfeldt-Jakob disease) [2] . Neuropathologically, prion diseases show widespread spongiosis, neuronal loss and gliosis with strain-specific patterns of neuronal cell tropism. The spread of misfolded prion protein throughout the brain from the site of initial prion conversion appears to be a process dependent on close cell association, often occurring along well-defined synaptic tracts [3] . There is growing evidence that several other proteinopathies that result in neurodegeneration may follow a similar prion-like spread of protein misfolding from a localized region, making the study of this process relevant to other diseases including Alzheimer's disease and Parkinson's disease [4] . Despite intense efforts, the cell biology of prion conversion and trafficking is relatively poorly defined. Cell lines that are susceptible to prion infection have been used to model the process in vitro [5] , [6] , [7] but are limited because the infectious agent PrP Sc is immunologically indistinguishable from the PrP C expressed on the recipient cell. This means that newly formed PrP Sc generated on the recipient cell cannot be specifically identified, making the conversion process itself difficult to study directly. Previous studies have relied on prolonged culture of cell lines that stably propagate prions to clear any inocula-derived PrP Sc —known to persist in cells for two weeks or more [8] , [9] —before the cell biology of newly formed PrP Sc can be analysed [10] . Therefore, fundamental information such as the timescale of the infection process or the cellular site in which the initial PrP conversion occurs has not been established. To study the earliest events in cellular prion infection, it is essential to distinguish the inocula-derived PrP Sc species from newly formed PrP Sc generated in the recipient cell. Inserting an epitope tag into the sequence of the endogenous PrP C such that the tag can be used to differentiate de novo formed PrP Sc is an elegant solution to this problem; however, the generation of true infectious prions containing an epitope tag has yet to be demonstrated in cells. This is probably because the sequence sensitivity of the conversion process prevents the misfolding of most tagged PrP C molecules [11] . The sequence sensitivity is such that the prion seed (exogenous PrP Sc ) and PrP C substrate (endogenous cellular PrP C ) must have homologous primary structures for efficient conversion to take place, particularly in certain key regions of the PrP molecule [12] , [13] . Hence, previous attempts to produce PrP constructs with green fluorescent protein reporter inserts or other epitope tags have not generated PrP chimerae that are capable of prion conversion [14] , [15] . Here we report on the generation of a unique cell system in which a novel epitope-tagged PrP C is expressed in a neuroblastoma cell line in which the endogenous PrP C has been silenced by RNA interference. We show that this engineered PrP C chimera supports prion replication and results in the production of a bona fide epitope-tagged PrP Sc as evidenced by both in vitro assays and mice bioassays. Using this cellular system, we have studied the earliest events in cellular prion infection and PrP misfolding; we show that prion infection of cells is extremely rapid, occurring within 1 min of prion exposure, and demonstrate that the plasma membrane is the initial site of prion conversion. Generation of cell lines expressing epitope-tagged PrP Sc To study prion infection in cells expressing tagged PrP C constructs without any interference from the host wild-type PrP C , we produced PrP knockdown (KD) cells derived from the mouse PK1 prion-susceptible neuroblastoma cell line [16] , using RNA interference (RNAi) directed at the 3′ untranslated region (3′-UTR) of PrP C mRNA. This effectively silences PrP gene expression ( Fig. 1a,b ) and results in the complete inhibition of prion propagation ( Fig. 1c ). This strategy allows the expression of the mouse PrP C open reading frame from exogenous constructs lacking the 3′-UTR, and permits the expression of a panel of FLAG- and MYC-tagged PrP C chimerae. The PrP constructs were designed such that the epitope tags were inserted into regions of the murine PrP C sequence that are relatively unstructured, and therefore theoretically unlikely to interfere with prion conversion ( Supplementary Fig. S1a ) [12] , [17] . Wild-type PK1 cells, PrP-KD cells and cells expressing tagged PrP C constructs were exposed to Rocky Mountain Laboratory (RML) mouse prions, and their ability to support prion propagation was assayed using the Scrapie Cell Assay [16] . PrP constructs 22CysFLAG and 30GlyFLAG were found to reconstitute prion propagation very efficiently and contained high levels of PrP Sc . However, it became apparent during the course of our study that these amino (N)-terminal FLAG tags were readily cleaved during cellular processing such that a proportion of the tagged PrP Sc in the cells was not detected by the anti-FLAG antibodies, making them unsuitable for this study. Cells expressing PrP C with epitope tags placed centrally within the PrP sequence (for example, PrP-124AlaMYC, Supplementary Fig. S1a ) did not support prion propagation ( Fig. 1c ). However, cells expressing PrP-224AlaMYC with the epitope tag inserted near the carboxy (C)-terminus were found to propagate prions robustly and reproducibly ( Fig. 1c ). Immunofluorescence and immunoblot analyses demonstrate that the expression levels and the cellular distribution of PrP-224AlaMYC were similar to that of wild-type PrP C in PK1 cells ( Fig. 1a,b ). Immunoblotting of proteinase K (PK)-digested cell lysates from RML prion-infected PrP-224AlaMYC cells demonstrates that they contain protease-resistant PrP, a characteristic feature of PrP Sc [18] ( Supplementary Fig. S1b ). 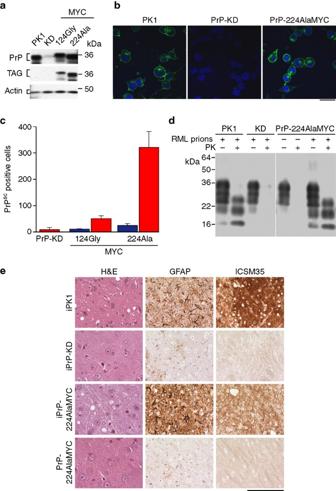Figure 1: Generation of prion-susceptible cell lines expressing epitope-tagged PrPCand PrPSc. (a) Western blots developed with anti-PrP and anti-MYC antibodies showing levels of PrPCin PK1, PrP-KD, PrP-124GlyMYC and PrP-224AlaMYC cell extracts. Actin is used as a loading control. Quantitative densitometry of similar blots that showed PrP expression was reduced by 90–95% in our PrP-KD cells. (b) Merged confocal images of PK1, PrP-KD and PrP-224AlaMYC cells stained with anti-PrP antibodies (green) and counterstained with 6-diamidino-2-phenylindole (blue) are shown; scale bar, 20 μm. (c) Scrapie Cell Assay (SCA) data showing the relative prion susceptibility of cell lines expressing PrP-MYC constructs compared with PrP-KD cells. Cells exposed to RML prions (red bars) or control cells (blue bars) were processed for the SCA. PrP molecules with the MYC tag inserted near the C-terminus at Ala224 support prion propagation; 124GlyMYC cells, uninfected PrP-224AlaMYC cells and infected PrP-KD cells do not contain PrPSc. The mean±s.e.m. of six independent experiments are shown. (d) Tg20 mice inoculated intracerebrally with extracts of prion-infected PrP-224AlaMYC cells develop prion disease. Western blots developed with anti-PrP antibodies showing that tg20 mice inoculated with extracts of prion-infected PK1 and PrP-224AlaMYC cells generate PK-resistant PrP (PrPSc) with a triplet band pattern similar to that of RML prions. (e) Histological analysis of tg20 mice brains inoculated with extracts of RML prion-infected PK1 cells (iPK1) and PrP-224AlaMYC cells (iPrP-224AlaMYC) revealed classical prion neuropathology with PrPScdeposition (ICSM35 immunostaining), neuronal loss and spongiosis (hematoxylin and eosin, H&E staining) and gliosis (GFAP immunostaining). Brains from animals inoculated with extracts of RML prion-infected PrP-KD cells (iPrP-KD) or control uninfected PrP-224AlaMYC cells (PrP-224AlaMYC) did not contain PrPScor show other diagnostic features. Scale bar is 80 μm on the H&E stained sections and 160 μm for all other panels. Figure 1: Generation of prion-susceptible cell lines expressing epitope-tagged PrP C and PrP Sc . ( a ) Western blots developed with anti-PrP and anti-MYC antibodies showing levels of PrP C in PK1, PrP-KD, PrP-124GlyMYC and PrP-224AlaMYC cell extracts. Actin is used as a loading control. Quantitative densitometry of similar blots that showed PrP expression was reduced by 90–95% in our PrP-KD cells. ( b ) Merged confocal images of PK1, PrP-KD and PrP-224AlaMYC cells stained with anti-PrP antibodies (green) and counterstained with 6-diamidino-2-phenylindole (blue) are shown; scale bar, 20 μm. ( c ) Scrapie Cell Assay (SCA) data showing the relative prion susceptibility of cell lines expressing PrP-MYC constructs compared with PrP-KD cells. Cells exposed to RML prions (red bars) or control cells (blue bars) were processed for the SCA. PrP molecules with the MYC tag inserted near the C-terminus at Ala224 support prion propagation; 124GlyMYC cells, uninfected PrP-224AlaMYC cells and infected PrP-KD cells do not contain PrP Sc . The mean±s.e.m. of six independent experiments are shown. ( d ) Tg20 mice inoculated intracerebrally with extracts of prion-infected PrP-224AlaMYC cells develop prion disease. Western blots developed with anti-PrP antibodies showing that tg20 mice inoculated with extracts of prion-infected PK1 and PrP-224AlaMYC cells generate PK-resistant PrP (PrP Sc ) with a triplet band pattern similar to that of RML prions. ( e ) Histological analysis of tg20 mice brains inoculated with extracts of RML prion-infected PK1 cells (iPK1) and PrP-224AlaMYC cells (iPrP-224AlaMYC) revealed classical prion neuropathology with PrP Sc deposition (ICSM35 immunostaining), neuronal loss and spongiosis (hematoxylin and eosin, H&E staining) and gliosis (GFAP immunostaining). Brains from animals inoculated with extracts of RML prion-infected PrP-KD cells (iPrP-KD) or control uninfected PrP-224AlaMYC cells (PrP-224AlaMYC) did not contain PrP Sc or show other diagnostic features. Scale bar is 80 μm on the H&E stained sections and 160 μm for all other panels. Full size image PrP-224AlaMYC cells propagate infectious tagged prions in vivo To confirm that our infected PrP-224AlaMYC cells were generating bona fide prions, the infectious nature of the 224-AlaMYC-PrP Sc was analysed in tg20 mice, a transgenic mouse line that overexpresses PrP often used in prion bioassays [19] . The mice were inoculated intracerebrally with extracts from RML prion-infected PrP-224AlaMYC-expressing cells. PK1 and PrP-KD cells infected in parallel with these cultures were used as positive and negative controls, respectively. Importantly, inoculation of tg20 mice with extracts from RML prion-infected PrP-KD cells (that do not propagate prions) did not result in prion disease in the mice ( Fig. 1d,e and Table 1 ). Inoculation of tg20 mice with RML prion-infected PrP-224AlaMYC cell extracts resulted in early clinical signs of scrapie, whereas extracts from control PrP-224AlaMYC cultures that were not previously exposed to RML prions did not ( Table 1 ). Biochemical analysis of the brains of the scrapie-affected mice showed that they contained PK-resistant PrP Sc ( Fig. 1d ). Histological analyses revealed classical prion neuropathology with PrP deposition, neuronal loss, spongiosis and gliosis ( Fig. 1e ). Control animals killed in parallel with the scrapie-affected mice did not contain PrP Sc or show any pathological features ( Fig. 1d,e ). These experiments demonstrate that our PrP-KD cells expressing PrP-224AlaMYC propagate true infectious tagged prions following RML prion exposure, and cause disease indistinguishable from that caused by RML prions propagated in wild-type PK1 cells. Table 1 In vivo bioassay of the infectious properties of the novel tagged-PrP molecules generated in PrP-224AlaMYC cells. Full size table Characterization of MYC-tagged PrP Sc cellular distribution To perform a detailed analysis of prion infection in cultured cells, it is necessary to distinguish newly synthesized PrP Sc from the host cellular PrP C . Three established methods achieve this by utilizing the biochemical differences between native PrP C and misfolded PrP Sc : These are PK digestion, guanidinium hydrochloride (GdnHCl) denaturation and formic acid extraction [20] , [21] . We compared each method in detail by immunostaining our PrP-224AlaMYC-expressing cells with anti-MYC antibodies. Both PK and formic acid treatment revealed a population of PK and formic acid-resistant MYC-tagged PrP Sc in prion-infected cells ( Fig. 2a,b ), with a strong signal at the plasma membrane and in the perinuclear compartment (PNC), consistent with previous observations of the sub-cellular distribution of PrP Sc (refs 20 , 22 , 23 ). In contrast, only very low levels of background immunostaining were detected in uninfected cells, indicating that PrP C had been effectively removed by these treatments. GdnHCl denaturation was less effective at removing PrP C staining ( Fig. 2a,b ). Similar results were obtained using ScPK1 cells that express wild-type PrP Sc (ref. 20 ) ( Supplementary Fig. S2a,b ), indicating that our MYC-tagged PrP Sc displays a physiologically relevant cellular localization. 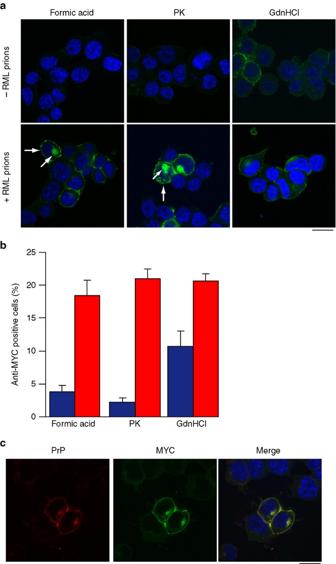Figure 2: Characterization ofde novoMYC-tagged PrPScdistribution in RML prion-infected cells. (a) Comparison of the methods used to visualize PrPScin RML prion-infected cells. Uninfected PrP-224AlaMYC cells (top panels) or chronically RML prion-infected PrP-224AlaMYC cells (passage five following prion exposure—bottom panels) were fixed and treated with 98% formic acid, proteinase K (PK) or guanidinium hydrochloride (GdnHCl) before staining with anti-MYC antibodies (green) and counterstaining with 6-diamidino-2-phenylindole (DAPI, blue). Merged confocal images are shown; scale bar, 20 μm. A proportion of the RML prion-infected cells contain formic acid and PK-resistant PrP (PrPSc) with a characteristic plasma membrane/perinuclear compartment distribution (arrow). (b) Quantification of randomly chosen cell fields from uninfected PrP-224AlaMYC cells (blue bars) or chronically RML prion-infected PrP-224AlaMYC cells (red bars). Approximately 20% of the cells in cultures exposed to RML prions contain formic acid/PK-resistant PrP (PrPSc). The background staining observed in the uninfected PrP-224AlaMYC cells after formic acid and PK treatment is mostly attributable to clumped cells in which access to the PrPCis restricted. The mean±s.e.m. from four independent experiments are shown. (c) Chronically RML prion-infected PrP-224AlaMYC cells were fixed and treated with 98% formic acid before staining with anti-MYC antibodies (green) and anti-PrP antibodies (red); the cells were counterstained with DAPI (blue). Single channels and merged confocal images are shown as indicated; scale bar, 20 μm. Figure 2: Characterization of de novo MYC-tagged PrP Sc distribution in RML prion-infected cells. ( a ) Comparison of the methods used to visualize PrP Sc in RML prion-infected cells. Uninfected PrP-224AlaMYC cells (top panels) or chronically RML prion-infected PrP-224AlaMYC cells (passage five following prion exposure—bottom panels) were fixed and treated with 98% formic acid, proteinase K (PK) or guanidinium hydrochloride (GdnHCl) before staining with anti-MYC antibodies (green) and counterstaining with 6-diamidino-2-phenylindole (DAPI, blue). Merged confocal images are shown; scale bar, 20 μm. A proportion of the RML prion-infected cells contain formic acid and PK-resistant PrP (PrP Sc ) with a characteristic plasma membrane/perinuclear compartment distribution (arrow). ( b ) Quantification of randomly chosen cell fields from uninfected PrP-224AlaMYC cells (blue bars) or chronically RML prion-infected PrP-224AlaMYC cells (red bars). Approximately 20% of the cells in cultures exposed to RML prions contain formic acid/PK-resistant PrP (PrP Sc ). The background staining observed in the uninfected PrP-224AlaMYC cells after formic acid and PK treatment is mostly attributable to clumped cells in which access to the PrP C is restricted. The mean±s.e.m. from four independent experiments are shown. ( c ) Chronically RML prion-infected PrP-224AlaMYC cells were fixed and treated with 98% formic acid before staining with anti-MYC antibodies (green) and anti-PrP antibodies (red); the cells were counterstained with DAPI (blue). Single channels and merged confocal images are shown as indicated; scale bar, 20 μm. Full size image The distribution of the formic acid-resistant MYC-tagged PrP Sc in PrP-224AlaMYC cells was analysed in detail by dual staining of formic acid-treated cells with anti-MYC and anti-PrP antibodies; importantly, anti-MYC and anti-PrP antibody staining colocalized ( Fig. 2c ). Further, dual staining experiments using anti-MYC antibodies and antibodies directed against various intracellular markers show partial colocalization of these compartments with formic acid-resistant MYC-tagged PrP Sc ( Supplementary Fig. S3 ), consistent with previous reports [7] , [20] , [22] , [24] and validating the use of formic acid treatment to reveal PrP Sc in cultured cells. MYC-tagged PrP Sc is rapidly formed following prion exposure Our novel cell system expressing MYC-tagged PrP Sc combined with effective PrP C removal by formic acid or PK treatment allows de novo synthesized PrP Sc to be clearly distinguished from the host RML prion inocula. This makes a detailed temporal and spatial study of the early stages of cellular prion infection feasible. Previous work in the field suggests that a 72-h exposure to prion-infected material is necessary to fully infect susceptible cells [16] . Therefore, we first infected PrP-224AlaMYC cells with RML prions for 3 days, and either fixed immediately or passaged in fresh media before fixation, formic acid extraction and anti-MYC staining. Maximum numbers of RML prion-infected MYC-tagged PrP Sc cells were seen 6 days post infection (DPI; Fig. 3a ) and stable prion propagation in ∼ 20% of the cells was observed up to 14 DPI ( Fig. 3a ). PrP-KD cells treated in the same way showed no anti-MYC immunostaining up to 6 DPI ( Fig. 3a ), indicating that the observed staining was dependent on PrP-224AlaMYC expression. Interestingly, a significant proportion of the PrP-224AlaMYC cells already contained MYC-tagged PrP Sc after 3 days of RML prion exposure ( Fig. 3a ). This prompted us to examine the first 72 h of prion exposure in more detail. 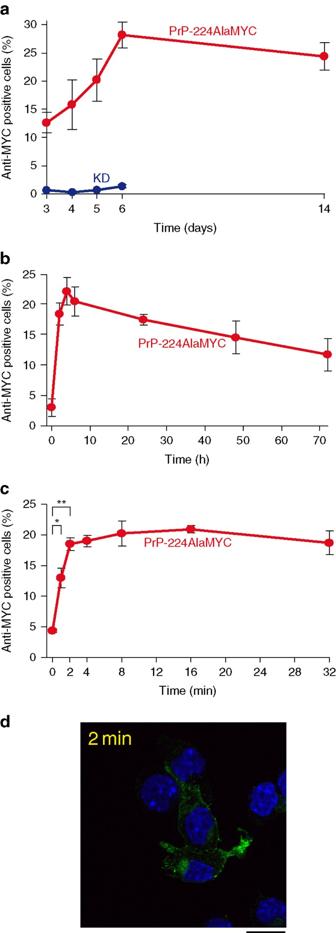Figure 3: MYC-tagged PrPScis synthesized rapidly, following RML prion exposure. (a) PrP-224AlaMYC cells were exposed to RML prions for 72 h, then fixed immediately or washed and cultured in fresh media (without RML prions) for the indicated durations before fixation and formic acid extraction. The proportion of anti-MYC-positive (RML prion infected) cells fixed at the indicated durations was quantified (red). As a control, PrP-KD cells were exposed to RML prions and processed in parallel (blue). The mean±s.e.m. from four independent experiments are shown. (b) PrP-224AlaMYC cells were exposed to RML prions for 0–72 h, then fixed and extracted with formic acid. The proportion of anti-MYC-positive (RML prion infected) cells fixed at the indicated durations was quantified. The mean±s.e.m. from four independent experiments are shown. Before RML prion exposure (0 h), few PrP-positive cells are detected, whereas RML prion exposure causes the rapid build-up of formic acid-resistant PrP (PrPSc) detectable as early as 2 h or less. (c) PrP-224AlaMYC cells were exposed to RML prions for 0–32 min, then fixed and extracted with formic acid. The proportion of anti-MYC-positive (prion infected) cells fixed at the indicated durations was quantified. The mean±s.e.m. from four independent experiments are shown; at the 0-, 1- and 2-min time points, the mean±s.e.m. from eight experiments is shown (*P<0.05, **P<0.001, two-tailedt-test). (d) PrP-224AlaMYC cells were exposed to RML prions for 2 min, then fixed and digested with PK. A confocal image stained with anti-MYC antibodies (green) and counterstained with 6-diamidino-2-phenylindole (blue) is shown. PK-resistant PrP (that is, PrPSc) was generated after just 2 min of RML prion exposure; scale bar, 20 μm. Figure 3b shows the proportion of infected cells at different time points of RML prion exposure and reveals that PrP-224AlaMYC cells produce PrP Sc rapidly, with MYC-tagged PrP Sc -positive prion-infected cells clearly detectable after 2 h of RML prion exposure. These observations suggest that cellular prion infection is faster than previously thought. Therefore, we examined the first few minutes of prion exposure in more detail. PrP-224AlaMYC cells were exposed to RML prions for very short periods before rapid washing and fixation. A significant proportion of the cells showed clearly detectable levels of formic acid-resistant MYC-tagged PrP Sc after as little as 1 min of exposure to RML prions ( Fig. 3c ), the shortest time period technically possible to reproduce accurately within the limitations of our system. PK digestion of similar cells confirmed that protease-resistant MYC-tagged PrP Sc was generated after very short periods of prion exposure ( Fig. 3d ). Figure 3: MYC-tagged PrP Sc is synthesized rapidly, following RML prion exposure. ( a ) PrP-224AlaMYC cells were exposed to RML prions for 72 h, then fixed immediately or washed and cultured in fresh media (without RML prions) for the indicated durations before fixation and formic acid extraction. The proportion of anti-MYC-positive (RML prion infected) cells fixed at the indicated durations was quantified (red). As a control, PrP-KD cells were exposed to RML prions and processed in parallel (blue). The mean±s.e.m. from four independent experiments are shown. ( b ) PrP-224AlaMYC cells were exposed to RML prions for 0–72 h, then fixed and extracted with formic acid. The proportion of anti-MYC-positive (RML prion infected) cells fixed at the indicated durations was quantified. The mean±s.e.m. from four independent experiments are shown. Before RML prion exposure (0 h), few PrP-positive cells are detected, whereas RML prion exposure causes the rapid build-up of formic acid-resistant PrP (PrP Sc ) detectable as early as 2 h or less. ( c ) PrP-224AlaMYC cells were exposed to RML prions for 0–32 min, then fixed and extracted with formic acid. The proportion of anti-MYC-positive (prion infected) cells fixed at the indicated durations was quantified. The mean±s.e.m. from four independent experiments are shown; at the 0-, 1- and 2-min time points, the mean±s.e.m. from eight experiments is shown (* P <0.05, ** P <0.001, two-tailed t -test). ( d ) PrP-224AlaMYC cells were exposed to RML prions for 2 min, then fixed and digested with PK. A confocal image stained with anti-MYC antibodies (green) and counterstained with 6-diamidino-2-phenylindole (blue) is shown. PK-resistant PrP (that is, PrP Sc ) was generated after just 2 min of RML prion exposure; scale bar, 20 μm. Full size image Further experiments ( Supplementary Fig. S4 ) confirmed that prion infection is rapid in our system. Washing the cells to remove inocula before culturing the cells in the fresh media (without inocula), demonstrated that short periods of RML prion exposure are sufficient to generate stable PrP Sc propagation in our cells. Quantifying the anti-MYC label incorporated into PrP-224AlaMYC cells following RML prion exposure showed that MYC-tagged PrP Sc builds up rapidly, reaching maximium levels by 2 h, which are maintained for at least 24 h. We also found that the proportion of prion-susceptible PrP-224AlaMYC cells was not increased if higher concentrations of inocula were applied. Prion conversion occurs at the cell surface within 1 min The steep rise in the number of prion-infected cells observed in the first 2 min following RML prion exposure indicates that this is the period when most cells first begin to synthesize PrP Sc ( Fig. 3c ). This allowed us to study the cellular site of this initial prion conversion. Examination of cells that were fixed after 1 min of prion exposure revealed that the MYC-tagged PrP Sc signal is only present at the plasma membrane. Orthogonal projections of serial confocal sections clearly showed that PrP Sc is present only at the cell surface ( Fig. 4a —1 min, white arrows—the z stack series is shown in Supplementary Fig. S5a ). This cellular distribution is strikingly different from the more typical plasma membrane and intracellular localization observed in cells that have been exposed to RML prions for longer durations ( Fig. 4a —180 min, arrows—the z stack series is shown in Supplementary Fig. S5b ). Categorizing the cells into three phenotypes of different PrP Sc distributions (plasma membrane, plasma membrane/diffuse intracellular and plasma membrane/PNC), and examining each phenotype at different durations following RML prion exposure revealed a rapid transition from the plasma membrane distribution seen at the earliest time point to the typical plasma membrane/PNC distribution observed later ( Fig. 4b ). Indeed, cells showing exclusively plasma membrane MYC-tagged PrP Sc staining disappeared after 2 min of exposure to RML prions, consistent with rapid PrP Sc formation, endocytosis and trafficking. 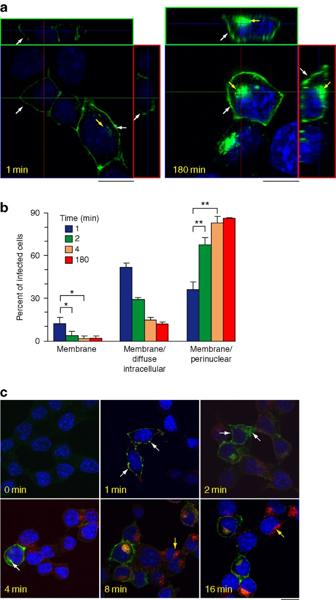Figure 4: Prion conversion first occurs at the cell surface within 1 min of prion exposure. (a) PrP224-AlaMYC cells were exposed to RML prions for the indicated durations, and then fixed and extracted with formic acid before staining with anti-MYC antibodies (green) and counterstaining with 6-diamidino-2-phenylindole (DAPI, blue). Orthogonal projections (red and green squares) of serial confocal sections are shown alongside one z-section taken from the middle of the cell (as indicated by the guidelines). A cell fixed after a 1-min exposure to RML prions shows PrPScimmunostaining only at the cell surface (1 min, white arrow). An adjacent cell in the field that has high levels of plasma membrane PrPScalso shows low intracellular levels of PrPSc(1 min, yellow arrow). Cells exposed to RML prions for 180 min show the typical steady-state distribution of PrPSc, with strong immunostaining at the plasma membrane (white arrows) and in the perinuclear region (yellow arrow −180 min); scale bar, 10 μm. (b) Quantification of cell phenotypes observed at different time points following prion exposure (the mean±s.e.m. from four independent experiments are shown; *P<0.05, **P<0.01, two-tailedt-test. The exactP-values are: membrane 1–2 min, 0.022; membrane 1–4 min, 0.049; membrane/PNC 1–2 min, 0.0049; membrane PNC 1–4 min, 0.0057). (c) PrP-224AlaMYC cells were exposed to RML prions and Texas red-labelled transferrin (red) for the indicated durations, then fixed and extracted with formic acid. Merged confocal images of cells stained with anti-MYC antibodies (green) and counterstained with DAPI (blue) are shown; scale bar, 20 μm. Initially, PrPScshows a plasma membrane distribution (1 min, arrows) and/or diffuse intracellular distribution (2 min, arrows) and then rapidly attains its steady-state distribution concentrated at the plasma membrane and PNC (4 min, white arrow indicates strong PNC stain). Initially, transferrin could be observed in small puncta at the cell periphery, reaching its equilibrium distribution in recycling endosomes at the PNC (yellow arrows) between 8 and 16 min. Figure 4: Prion conversion first occurs at the cell surface within 1 min of prion exposure. ( a ) PrP224-AlaMYC cells were exposed to RML prions for the indicated durations, and then fixed and extracted with formic acid before staining with anti-MYC antibodies (green) and counterstaining with 6-diamidino-2-phenylindole (DAPI, blue). Orthogonal projections (red and green squares) of serial confocal sections are shown alongside one z-section taken from the middle of the cell (as indicated by the guidelines). A cell fixed after a 1-min exposure to RML prions shows PrP Sc immunostaining only at the cell surface (1 min, white arrow). An adjacent cell in the field that has high levels of plasma membrane PrP Sc also shows low intracellular levels of PrP Sc (1 min, yellow arrow). Cells exposed to RML prions for 180 min show the typical steady-state distribution of PrP Sc , with strong immunostaining at the plasma membrane (white arrows) and in the perinuclear region (yellow arrow −180 min); scale bar, 10 μm. ( b ) Quantification of cell phenotypes observed at different time points following prion exposure (the mean±s.e.m. from four independent experiments are shown; * P <0.05, ** P <0.01, two-tailed t -test. The exact P -values are: membrane 1–2 min, 0.022; membrane 1–4 min, 0.049; membrane/PNC 1–2 min, 0.0049; membrane PNC 1–4 min, 0.0057). ( c ) PrP-224AlaMYC cells were exposed to RML prions and Texas red-labelled transferrin (red) for the indicated durations, then fixed and extracted with formic acid. Merged confocal images of cells stained with anti-MYC antibodies (green) and counterstained with DAPI (blue) are shown; scale bar, 20 μm. Initially, PrP Sc shows a plasma membrane distribution (1 min, arrows) and/or diffuse intracellular distribution (2 min, arrows) and then rapidly attains its steady-state distribution concentrated at the plasma membrane and PNC (4 min, white arrow indicates strong PNC stain). Initially, transferrin could be observed in small puncta at the cell periphery, reaching its equilibrium distribution in recycling endosomes at the PNC (yellow arrows) between 8 and 16 min. Full size image To confirm this result, we directly compared the formation and trafficking of MYC-tagged PrP Sc to the endocytosis of Texas red-labelled transferrin. Transferrin endocytosis and trafficking occurs rapidly, reaching a steady-state distribution at the PNC between 8 and 16 min [25] ( Fig. 4c ). In the same cells, PrP Sc attained a steady-state distribution in nearly all cells by 4 min of exposure to prions ( Fig. 4b,c ). Therefore, prion protein conversion and endocytosis proceeds at rates that are similar to that of transferrin trafficking. To determine whether PrP prion conversion can occur on the plasma membrane, we incubated pre-cooled PrP-224AlaMYC cells with RML prions at 4 °C. This temperature shift effectively abolished endocytosis in mammalian cells [26] . Significantly, PrP Sc accumulated only on the cell surface under these conditions ( Fig. 5a,b , 4 °C). Orthogonal projections of confocal sections taken through these infected cells revealed the plasma membrane distribution of MYC-tagged PrP Sc ( Fig. 5a —the z stack series is shown in Supplementary Fig. S6 ) and clearly demonstrated that endocytosis is not necessary to produce misfolded PrP. 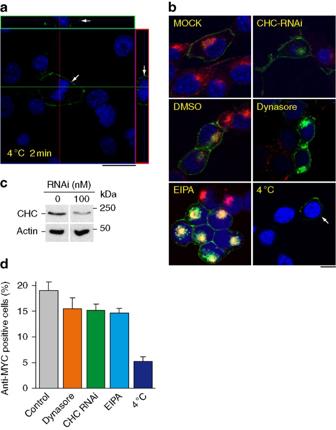Figure 5: PrPScforms at the cell surface. (a) Pre-cooled PrP-224AlaMYC cells were exposed to RML prions for 2 min on ice, then fixed and extracted with formic acid. Orthogonal reconstructions of serial confocal slices are shown (red and green boxes) alongside one z-slice taken from near the middle of the cells (as indicated by the guide lines). The cells were fixed after 2 min and stained with anti-MYC antibodies (green) and counterstained with 6-diamidino-2-phenylindole (DAPI, blue); scale bar, 20 μm. Formic acid-resistant PrP (PrPSc) is formed on the cell surface of one of the cells in the field (arrow), no intracellular PrPScwas detected. (b) PrP-224AlaMYC cells were mock-transfected or transfected with RNAi directed at CHC, pretreated with dynasore (80 μM), EIPA (100 μM) or pre-cooled to 4 °C. RML prions were added in the continued presence of the treatments for 180 min and Texas red-labelled transferrin (red) was added for the final 10 min of incubation. The cells were then fixed and extracted with formic acid. Merged confocal images of cells stained with anti-MYC antibodies (green) and counterstained with DAPI (blue) are shown; scale bar, 20 μm. Following prion exposure at 4 °C, MYC-tagged PrPScwas detected only at the plasma membrane (arrow). (c) Lysates from PrP-224AlaMYC cells mock-transfected or transfected with RNAi directed at CHC were collected and subjected to SDS–polyacrylamide gel electrophoresis. Immunoblots developed with anti-CHC and anti-actin antibodies are shown. Quantitative densitometry of similar blots showed that CHC expression was reduced by∼70% in the RNAi-treated cells. (d) PrP-224AlaMYC cells were treated as inb. The percentage of anti-MYC-positive (RML prion infected) cells observed was quantified for each condition. The mean±s.e.m. from three independent experiments are shown (background levels found in uninfected cells for each condition have been subtracted from the mean). Figure 5: PrP Sc forms at the cell surface. ( a ) Pre-cooled PrP-224AlaMYC cells were exposed to RML prions for 2 min on ice, then fixed and extracted with formic acid. Orthogonal reconstructions of serial confocal slices are shown (red and green boxes) alongside one z-slice taken from near the middle of the cells (as indicated by the guide lines). The cells were fixed after 2 min and stained with anti-MYC antibodies (green) and counterstained with 6-diamidino-2-phenylindole (DAPI, blue); scale bar, 20 μm. Formic acid-resistant PrP (PrP Sc ) is formed on the cell surface of one of the cells in the field (arrow), no intracellular PrP Sc was detected. ( b ) PrP-224AlaMYC cells were mock-transfected or transfected with RNAi directed at CHC, pretreated with dynasore (80 μM), EIPA (100 μM) or pre-cooled to 4 °C. RML prions were added in the continued presence of the treatments for 180 min and Texas red-labelled transferrin (red) was added for the final 10 min of incubation. The cells were then fixed and extracted with formic acid. Merged confocal images of cells stained with anti-MYC antibodies (green) and counterstained with DAPI (blue) are shown; scale bar, 20 μm. Following prion exposure at 4 °C, MYC-tagged PrP Sc was detected only at the plasma membrane (arrow). ( c ) Lysates from PrP-224AlaMYC cells mock-transfected or transfected with RNAi directed at CHC were collected and subjected to SDS–polyacrylamide gel electrophoresis. Immunoblots developed with anti-CHC and anti-actin antibodies are shown. Quantitative densitometry of similar blots showed that CHC expression was reduced by ∼ 70% in the RNAi-treated cells. ( d ) PrP-224AlaMYC cells were treated as in b . The percentage of anti-MYC-positive (RML prion infected) cells observed was quantified for each condition. The mean±s.e.m. from three independent experiments are shown (background levels found in uninfected cells for each condition have been subtracted from the mean). Full size image To test this hypothesis, we used a range of pharmacological and genetic manipulations designed to inhibit the endocytic pathways that were previously implicated in prion metabolism—dynamin- and clathrin-dependent endocytosis and macropinocytosis. Dynasore was used as a direct dynamin inhibitor [27] and RNAi directed at the clathrin heavy chain (CHC) was used to interfere with clathrin function. The functional efficacy of both treatments was shown by the reduced labelled transferrin uptake in the cells, a well-characterized cargo for dynamin- and clathrin-dependent endocytosis ( Fig. 5b ). Immunoblotting showed that RNAi treatment effectively reduced overall CHC levels ( Fig. 5c ). However, the transfection efficiency of the RNAi delivery varied in our cell population, with some cells showing an almost complete block in transferrin uptake and other cells maintaining residual endocytic capacity ( Fig. 5b ). Dynasore and RNAi directed at the CHC did not significantly affect RML prion infection or PrP Sc internalization ( Fig. 5b,d ), and no correlation was observed between an individual cell's susceptibility to prion infection and its ability to endocytose transferrin. Macropinocytosis was targeted using the ion transport inhibitor ( N -ethyl- N -isopropyl)amiloride (EIPA) [28] . This treatment had no effect on labelled transferrin uptake and did not affect RML prion infection in our system ( Fig. 5b,d ). Incubating pre-cooled PrP-224AlaMYC cells with RML prions at 4 °C confirms that blocking all endocytosis—demonstrated by the lack of transferrin uptake—does not ablate prion conversion ( Fig. 5b,d ). An important role for plasma membrane PrP C expression in prion conversion was confirmed by experiments using phosphoinositide-specific phospholipase C (PIPLC) to deplete plasma membrane PrP C . This significantly reduced the generation of MYC-tagged PrP Sc ( Fig. 6a,b ). It is interesting to note that many of the cells in the PrP-224AlaMYC cultures bind and/or internalize inocula-derived PrP Sc following RML prion exposure, independent of surface PrP C expression ( Fig. 6a ). Further, striking examples of this phenomenon are included in Supplementary Figure S7 . This suggests that other factors in addition to a simple physical association of cellular PrP C with PrP Sc affect prion conversion, an observation in agreement with previously published data [29] , [30] , [31] . 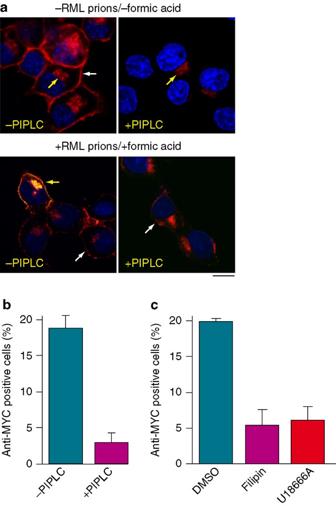Figure 6: Plasma membrane PrPCis required for efficient prion infection. (a) Upper panel: PrP-224AlaMYC cells were treated with PIPLC (0.5 U ml−1) for 2 h before fixation and immunostaining with anti-PrP antibodies (red) and counter staining with 6-diamidino-2-phenylindole (DAPI, blue). Merged confocal images are shown; scale bar, 20 μm. Control cells (−PIPLC) show strong plasma membrane (white arrow) and intracellular (yellow arrow) PrP immunostaining. PIPLC effectively removed surface plasma membrane-bound PrP (+PIPLC), but residual intracellular PrP immunostaining was seen (yellow arrow). Lower panel: Untreated and PIPLC-treated PrP224AlaMYC cells were exposed to RML prions for 180 min, then fixed and extracted with formic acid. Merged confocal images of cells stained with anti-MYC (green) and anti-PrP antibodies (red), then counterstained with DAPI (blue) are shown; scale bar, 20 μm. Formic acid-resistant PrPScderived from the inocula and immunostained with anti-PrP antibodies only (red) can be seen closely associated with all the cells independent of PIPLC treatment (examples are indicated by white arrows). One untreated cell (−PIPLC, yellow arrow) in the field shown has generatedde novoMYC-tagged PrPScas indicated by anti-MYC (green) and anti-PrP (red) immunostaining, which appears yellow in the merged image. No cells have generated MYC-tagged PrPScfollowing PIPLC treatment (+PIPLC). (b) PrP-224AlaMYC cells were treated as inFigure 6alower panel. The percentage of anti-MYC-positive (RML prion infected) cells was quantified for each condition. The mean±s.e.m. from three independent experiments are shown (background levels found in uninfected cells for each condition have been subtracted from the mean). (c) PrP-224AlaMYC cells were pretreated with vehicle (DMSO) or filipin (5 μg ml−1) for 30 min, or U18666A (1 μg ml−1) for 16 h, then exposed to RML prions for 180 min in the continued presence of the vehicle or inhibitor. Cells were then fixed and extracted with formic acid before immunostaining with anti-MYC antibodies. The percentage of anti-MYC-positive (RML prion-infected) cells was quantified. The mean±s.e.m. from three independent experiments are shown (background levels found in uninfected cells for each condition for have been subtracted from the mean). Figure 6: Plasma membrane PrP C is required for efficient prion infection. ( a ) Upper panel: PrP-224AlaMYC cells were treated with PIPLC (0.5 U ml −1 ) for 2 h before fixation and immunostaining with anti-PrP antibodies (red) and counter staining with 6-diamidino-2-phenylindole (DAPI, blue). Merged confocal images are shown; scale bar, 20 μm. Control cells (−PIPLC) show strong plasma membrane (white arrow) and intracellular (yellow arrow) PrP immunostaining. PIPLC effectively removed surface plasma membrane-bound PrP (+PIPLC), but residual intracellular PrP immunostaining was seen (yellow arrow). Lower panel: Untreated and PIPLC-treated PrP224AlaMYC cells were exposed to RML prions for 180 min, then fixed and extracted with formic acid. Merged confocal images of cells stained with anti-MYC (green) and anti-PrP antibodies (red), then counterstained with DAPI (blue) are shown; scale bar, 20 μm. Formic acid-resistant PrP Sc derived from the inocula and immunostained with anti-PrP antibodies only (red) can be seen closely associated with all the cells independent of PIPLC treatment (examples are indicated by white arrows). One untreated cell (−PIPLC, yellow arrow) in the field shown has generated de novo MYC-tagged PrP Sc as indicated by anti-MYC (green) and anti-PrP (red) immunostaining, which appears yellow in the merged image. No cells have generated MYC-tagged PrP Sc following PIPLC treatment (+PIPLC). ( b ) PrP-224AlaMYC cells were treated as in Figure 6a lower panel. The percentage of anti-MYC-positive (RML prion infected) cells was quantified for each condition. The mean±s.e.m. from three independent experiments are shown (background levels found in uninfected cells for each condition have been subtracted from the mean). ( c ) PrP-224AlaMYC cells were pretreated with vehicle (DMSO) or filipin (5 μg ml −1 ) for 30 min, or U18666A (1 μg ml −1 ) for 16 h, then exposed to RML prions for 180 min in the continued presence of the vehicle or inhibitor. Cells were then fixed and extracted with formic acid before immunostaining with anti-MYC antibodies. The percentage of anti-MYC-positive (RML prion-infected) cells was quantified. The mean±s.e.m. from three independent experiments are shown (background levels found in uninfected cells for each condition for have been subtracted from the mean). Full size image Rapid prion conversion on the cell surface may point to a mechanism in which PrP misfolding is a stochastic event catalysed by the interaction with PrP Sc in a favourable environment such as that found in lipid rafts, membrane microdomains thought to have a role in prion conversion [32] . We therefore tested whether reagents that disrupt lipid raft integrity would affect prion protein conversion. Two reagents that affect lipid raft function by different mechanisms—filipin [33] , which binds and sequesters plasma membrane cholesterol, and U18666A, which inhibits cholesterol transport to rafts [34] —abrogated prion conversion in our cellular system ( Fig. 6c ). We report on the generation of a unique cell system in which an epitope-tagged PrP C is expressed in a prion-susceptible neuroblastoma cell line in which the host PrP C has been removed using RNAi. This engineered PrP C was shown to support prion replication resulting in the production of a true bona fide , infectious epitope-tagged PrP Sc . Using this cellular system we have shown that prion infection of cells is extremely rapid, occurring within 1 min of prion exposure, and we demonstrate unequivocally that the plasma membrane is the initial site of prion conversion. Generating an epitope-tagged PrP C chimera that is capable of prion conversion and forming an infectious tagged PrP Sc is not straightforward. A C-terminal green fluorescent protein-tagged PrP C construct produced by Barmada and Harris [14] failed to form PrP Sc and even the insertion of a small 10-amino-acid MYC tag at ser-230 of murine PrP abrogated prion conversion when expressed in a PrP C knockout mouse background [15] . We designed a panel of eight different constructs based on a biophysical analysis of PrP C structure, and screened them for the ability to reconstitute prion propagation in our PrP-KD cells. In agreement with an earlier report [17] PrP constructs with FLAG tags inserted near the N-terminus supported efficient prion conversion, but could not be used because this region of the protein was cleaved during the cellular processing of PrP Sc . Epitope tags inserted into the central region of the PrP C molecule did not support prion propagation, consistent with previous reports on the importance of sequence conservation in this region for efficient conversion [12] , [13] . However, one of our constructs, PrP-224AlaMYC, robustly generated epitope-tagged PrP Sc . Significantly, a mouse bioassay demonstrated that the PrP-224AlaMYC cells propagate genuine infectious prions. The capacity of PrP-224AlaMYC cells to produce epitope-tagged PrP Sc , combined with effective protocols to remove PrP C from our cells, allowed us to examine PrP misfolding when prions initially contact and infect susceptible cells. Our temporal analysis of the events immediately following cellular prion exposure revealed that prion infection is far faster than previously thought. Earlier studies had indicated that PrP Sc /cell interactions may be rapid [35] , but de novo PrP Sc formation was not studied directly. Here we have demonstrated in a cellular system the rapid protein misfolding and aggregation observed in cell-free experiments [36] . Consistent with the highly dynamic nature of prion infection of PrP-224AlaMYC cells, we observed that PrP Sc had attained steady-state levels by 2 h following RML prion exposure and did not change significantly up to 24 h, indicating that PrP Sc metabolism is highly dynamic and the synthesis and breakdown appear normally balanced in these cells. A detailed spatial analysis of cells shortly after prion exposure demonstrated that PrP Sc forms on the plasma membrane. The plasma membrane has been suggested to be a potential site of PrP conversion [7] , [21] , [22] , [37] , which is consistent with the observed PrP Sc distribution reported in different cell and in vivo systems [21] , [24] , [38] . Our observations that prion conversion proceeds even at 4 °C under conditions that prohibit endocytic activity in mammalian cells [26] confirms that the plasma membrane alone is sufficient for the process. Supporting this idea, we have also shown that plasma membrane PrP C expression is required for efficient prion infection. PIPLC treatment effectively removed plasma membrane PrP C from PrP-224AlaMYC cells and greatly reduced the generation of PrP Sc . This is consistent with previous reports showing that PIPLC treatment reduced the generation of PrP Sc in chronically prion-infected PK1 cells [39] , and data indicating that PrP C lacking the GPI anchor (and hence not expressed on the cell surface) does not support efficient PrP Sc production or stable cellular prion infection [40] . The role of the plasma membrane in prion conversion was explored further by experimental treatments designed to inhibit dynamin/clathrin-dependent endocytosis and macropinocytosis, pathways that have been previously implicated in prion metabolism [35] , [41] . These manipulations had little effect on prion infection or PrP Sc internalization. This suggests that either they are not involved in PrP Sc internalization or that the process can occur through multiple pathways, an idea supported by the literature [32] . Our data also suggest that prion conversion is dependent on the presence of intact lipid rafts, specialized membrane microdomains known to be present in the plasma membrane and enriched in PrP C (refs 42 , 43 ). Supporting this idea, cofactors enriched in lipid rafts have been shown to stimulate synthetic prion conversion [29] , [31] and reagents that disrupt raft integrity abrogate PrP Sc propagation in cells [44] , [45] . Despite this, our data do not preclude a role for intracellular compartments in prion conversion, which may continue or accelerate the process following the endocytosis of PrP Sc . Previous reports have implicated various cell compartments in the conversion process [7] , [46] , [47] . Our observation that prion infection was reduced at 4 °C may reflect a slower reaction rate due to the lower temperature as might be expected for a protein-folding-driven phenomenon, but could also be consistent with an important role for internal compartments in PrP Sc propagation. As earlier studies relied on the analysis of cells already propagating prions that express intracellular PrP Sc before any manipulations designed to examine the region at which misfolding takes place [7] , [47] , [48] , the contribution of the plasma membrane to the initial prion conversion process may have been underestimated or overlooked. Our system has also allowed new insights into the dynamic nature of PrP Sc trafficking in the cell. The ability to analyse the trafficking events immediately following prion exposure has revealed that PrP Sc initially forms at the cell surface, and is rapidly endocytosed. Indeed, after 1 min of exposure to RML prions, many cells already contain intracellular PrP Sc , often in a diffuse cellular distribution, possibly reflecting a transition through an endosomal compartment. After 4 min of exposure to prions, PrP Sc takes up a steady-state distribution concentrated at the PNC and at the cell surface, as described in the literature [20] , [22] , [23] . The similarity in the appearance of these cells to cells that chronically propagate prions, and our data showing that a 2-min exposure to RML prion brain homogenate is sufficient to generate cells that continue to produce PrP Sc in the absence of further prion seed, suggests that cells are stably infected by prions in a very short time period. However, membrane binding and internalization of inocula-derived PrP Sc is not in itself sufficient to generate prion infection/ de novo PrP Sc production. This is clearly demonstrated by our novel cell system and suggests that cell factors, in addition to a simple physical interaction between PrP C and PrP Sc , are required for prion formation. This idea has been postulated previously [29] , [31] and is supported by our demonstration that increasing the concentration of inocula added to our PrP224AlaMYC cultures did not lead to an increase in the proportion of infected cells. This indicates that only a proportion of our cells contain/express the necessary susceptibility factors required for prion conversion. In conclusion, we have presented the generation of a unique cell system producing bona fide epitope-tagged PrP Sc , which was analysed using both in vitro and in vivo assays. By visualizing MYC-tagged PrP Sc , we have been able to study the earliest events in cellular prion conversion. We have shown that cellular prion infection is a dynamic process that occurs within 1 min of prion exposure, and that the plasma membrane is the primary site of prion conversion. These results have important implications for our understanding of the conversion and spread of prions in vivo . Once a sufficient seed of infectious prions has been established in the brain, our data suggest that prion cellular spread is likely to proceed far more rapidly than previously thought. These data cast new light on why prion infection can be very aggressive in vivo and can affect the whole neural axis in just a few weeks. Cell lines and DNA constructs All cells were cultured in OptiMEM, FCS (10%) and penicllin/streptomycin. Short interfering RNA sequences targeting the 3′-UTR of PrP C were cloned into the pSUPER.retro.puro expression vector (Oligoengine) and introduced into wild-type PK1 cells by retroviral transduction [49] . Stable PrP knockout clones ( Supplementary Fig. S1 ) were isolated and cultured in puromycin selection media. Tagged PrP constructs were generated by overlap extension PCR procedures using standard methods [50] (primer sequences available on request), subcloned into the pLNCX-retroviral vector and then sequenced (Clontech). These were introduced into PK1-KD cells by retroviral transduction [51] , and stable lines expressing the tagged PrP constructs were isolated and routinely cultured in dual selection media (puromycin and G418, Invitrogen). Cellular prion infection and PrP Sc analyses Brain homogenates were prepared from end-stage RML prion-infected CD-1 mice as a 10% homogenate in PBS [16] . These were diluted to 0.1% in media, and added to cells grown to 70% confluence that were seeded on poly- L -lysine-coated glass coverslips or plastic dishes. After prion incubation, cells were washed three times with warm PBS and fixed, collected for biochemical analysis or passaged in the ratio 1:8. The Scrapie Cell Assay was performed as described previously [16] . Cells were routinely prepared for immunofluorescence analysis by fixation in 3.7% paraformaldehyde for 12 min at 37 °C, and then washing in PBS. PrP Sc was revealed specifically by a 5-min pre-treatment with 98% formic acid to remove host PrP C (ref. 20 ). PK digestion and GdnHCl treatment to remove PrP C and expose PrP Sc were as described [21] . To further characterize prion infection, PrP-224AlaMYC cells were exposed to varying concentrations of RML prions for 180 min before fixation, or incubated with 0.1% RML prions for 2 min, washed three times and fixed immediately or incubated in fresh medium lacking prions for a further 48 h before fixation. In addition, cells were pretreated with vehicle, dynasore (80 μM—added in serum-free media), EIPA (100 μM) and filipin (5 μg ml −1 ) for 30 min, or U18666A (1 μg ml −1 ) for 16 h, and then exposed to RML prions. Cells were transfected with RNAi oligos using Fugene 6 reagent according to the manufacturer's instructions. A mixture of four RNAi oligos targeting CHC (Dharmacon on target plus kit) was added at 100 nM for 30 h before the addition of RML prions. PIPLC treatment was carried out using 0.5 U ml −1 PIPLC for 2 h before the addition of RML prions [39] . The cells were then incubated with RML prions for 180 min in the continued presence of the treatment. Texas red-labelled transferrin (Invitrogen) was added to the media at 5 μg ml −1 for the last 10 min of the incubation. Control experiments replicating the conditions for each treatment but lacking the active reagents were carried out to check that conditions outside our treatments did not affect prion infection. No significant differences were observed. In our 4 °C experiments ( Fig. 5a,b ), cells were pre-cooled on ice for 30 min before the addition of RML prions made up in ice-cold media. Cells were washed three times with ice-cold PBS, fixed on ice for 10 min and then transferred to 37 °C for a further 10 min before washing with PBS and further processing. Immunofluorescence analysis Formic acid-treated and -untreated cells were permeabilized with cold methanol for 10 min at −20 °C and then washed with PBS, before blocking with 10% horse serum and 1% BSA in TBS. Primary antibody incubations were performed overnight at 4 °C in TBS/1% BSA. Following extensive washing in TBS, samples were incubated with AlexaFluor 488 and 543-labelled secondary antibodies diluted in TBS/1% BSA, as appropriate, for 1 h at room temperature. Cells were thoroughly washed in TBS and mounted in Antifade media (DAKO) containing 1-μg ml −1 4′,6-diamidino-2-phenylindole. The primary antibodies used in this study are detailed in Supplementary Table S1 . Fluorescence images were acquired using a Zeiss LSM510 meta confocal microscope (Zeiss) with a plan-Apochromat' ×63/1.40 oil DIC objective. Control uninfected cells were processed for each experiment and LSM settings were chosen to produce minimal background staining. The same settings were used to examine all infected cells in that experiment. The extent of MYC label incorporated into the cells was determined using Volocity software (Improvision). At least 50 cells from three independent experiments were analysed per condition. Orthogonal projections were generated from z-stacks using Zeiss LSM software (Zeiss). To determine prion infection, at least 300 cells from eight randomly chosen fields were counted for each condition, and the proportion of cells showing PrP Sc immunostaining after PrP C removal was calculated. All experiments were performed by two independent investigators. Blinded analysis by a third investigator was also undertaken. For cell phenotypic analyses, z-stacks encompassing the entire cell were obtained and cells were grouped into one of three categories based on the localization of MYC-tagged PrP Sc : exclusively plasma membrane, plasma membrane/diffuse intracellular and plasma membrane/PNC. In each experiment, at least 50 cells were analysed for each condition. Inoculation of tg20 mice and neuropathological analysis Inocula were prepared from PK1, PrP-KD and PrP-224AlaMYC cell cultures exposed to prions for 72 h and sub-passaged five times 1:8 (ref. 16 ). Cells were harvested in sterile PBS, washed twice and then resuspended to 30 million cells per ml. Control PrP-224AlaMYC cells that were not exposed to prions were collected the same way. Inocula were stored in sterile vessels at −80 °C until use. Animals were cared for per institutional and Home Office regulations. For each of the test conditions, groups of five tg20 mice were inoculated intracerebrally with 30 μl of cell suspension. Animals were observed daily for clinical signs and culled on diagnosis of prion disease. Two animals that were not diagnosed with prion disease were culled in parallel with the diseased animals, and the remaining animals were culled 4 to 5 weeks after the last diseased animal was diagnosed. Brains were excised and examined by histopathology and western blotting [52] . Biochemical analysis Cell lysates were collected for biochemical analysis in PBS, washed and resuspended in a small volume of fresh PBS [52] , [53] . The cells were lysed by three freeze/thaw cycles and benzonase (50 U ml −1 , Merck) was added for 20 min at 4 °C. Protein concentrations in the lysates were determined by Bio-Rad assay (Bio-Rad). For PK treatments, the samples were diluted to 2 mg ml −1 in PBS and Triton X-100 (1%) and PK (5 or 2.5 μg ml −1 ) was added. Samples were digested for 30 min at 37 °C and digestion was terminated by the addition of phenylmethylsulphonyl fluoride to a 1-mM sample. Proteins were precipitated with cold methanol and resuspended in SDS sample buffer. SDS–polyacrylamide gel electrophoresis and immunoblotting were carried out as described previously [52] . Statistical analysis Data were expressed as mean plus standard error of the mean (s.e.m. ), unless otherwise stated. Data were compared by two-tailed t -tests and considered significantly different when P <0.05. Degree of significance is expressed as follows: P <0.05*; P <0.01**; unless otherwise specified. How to cite this article: Goold, R. et al . Rapid cell-surface prion protein conversion revealed using a novel cell system. Nat. Commun. 2:281 doi: 10.1038/ncomms1282 (2011).